Large indentation strain-stiffening in nanotwinned cubic boron nitride Recent experiments reported a substantial strengthening of cubic boron nitride by nanotwinning. This discovery raises fundamental questions about new atomistic mechanisms governing incipient plasticity in nanostructured strong covalent solids. Here we reveal an unusual twin-boundary dominated indentation strain-stiffening mechanism that produces a large strength enhancement at nanometer-scale twinning size where a strength reduction is normally expected due to the reverse Hall–Petch effect. First-principles calculations unveil significantly enhanced indentation shear strength in nanotwinned cubic boron nitride by bond rearrangement at the twin boundary under indentation compression and shear strains that produces especially strong stress response. This remarkable strain-stiffening mechanism offers fundamental insights for understanding the stress response of nanotwinned covalent solids under indentation. Strengthening materials by microstructural size reduction, known as the Hall–Petch effect [1] , [2] , is achieved through suppression of nucleation and motion of dislocations by grain boundaries. Below a threshhold size, however, a reverse Hall–Petch effect takes place when interactions at grain boundaries dominate plastic deformation, leading to reduced strength. These trends, which are widely regarded as universal rules for metals [3] and covalent solids [4] , [5] , are challenged by recently synthesized nanotwinned cubic boron nitride (nt-cBN) [6] that exhibits an extraordinary strengthening at a twinning size down to a few nanometers. Similar effects were also observed in metallic multi-layer composites where strengthening continues into the layer-thickness scale of a few nanometers and deviates significantly from the Hall–Petch law [7] , [8] . Here we report an unusual twin-boundary dominated strengthening mechanism explaining the surprisingly high Vickers hardness of nt-cBN up to 108 GPa (ref. 6 ). Quantum-mechanical calculations reveal that this large hardness increase comes from a shear strengthening by the compressive pressure at the twin boundary, giving rise to a large strain stiffening in nt-cBN [9] . This novel mechanism offers new fundamental insights for understanding the incipient plasticity in nanotwinned covalent solids and a new way to design superhard materials using various nanotwinning structures. In most materials, nanoscale twin boundaries (TBs) act like regular grain boundaries (GBs) in modifying the mechanical properties by blocking dislocation motions [10] , [11] , [12] , [13] , [14] , [15] . The much lower formation energy of TBs makes them more stable than GBs during structural deformation and, therefore, more effective in strengthening materials. For example, nanotwinned Cu (nt-Cu) exhibits much higher tensile strength compared with those of ultrafine-grained Cu [10] , [11] as the TB separation λ decreases (the Hall–Petch effect) to λ =15 nm. At further reduced λ , however, the tensile strength of nt-Cu decreases (the reverse Hall–Petch effect) when TB-associated mechanism or TB–GB interactions become dominant [15] . Interestingly, all the molecular dynamics (MD) studied nanostructured Cu samples show a maximum strength (2.5~3.7 GPa) that is lower than the ideal tensile strength (4.2 GPa) for single crystal Cu [16] , and the measured maximum strength (1.1 GPa) of nt-Cu [10] , [11] is lower than that predicted by MD simulations [12] , [13] , [14] , [15] . Similar results have been observed in covalent materials, such as strength enhancement by reducing grain size d down to 10 nm in cBN in the Hall–Petch regime [17] , [18] and strength reduction in nanostructured diamond with d <4.5 nm (refs 4 , 5 ) whose peak tensile and shear strengths only reach less than half the values for single crystal diamond [19] , [20] , which is attributed to the weak interactions associated with the irregular bonds at the boundaries between nanocrystallites, a typical GB-dominated reverse Hall–Petch effect. The situation is drastically different for nt-cBN, which at an ultrafine twining size λ =3.8 nm has a greatly enhanced Vickers indentation hardness (95~108 GPa) [6] that is almost twice the value for single crystal cBN [17] , [18] . This sharp contrast of a giant strength hardening in the classic reverse Hall–Petch regime, where a strength softening is normally expected, indicates a new mechanism governing the mechanical property of nt-cBN. It was found recently that twin interfaces in nano-grain diamond (ng-dia) can enhance its elastic constants [21] , [22] . The reported experiments and calculations showed, however, that the increase of the elastic constants, especially the shear modulus, induced by the twin interfaces in ng-dia is just a few percent [22] , which is too small to explain the nearly 100% increase of hardness observed in nt-cBN [6] . Here we use first-principles calculations to determine the stress–strain relation of nt-cBN with twining sizes less than a few nanometers, and the obtained indentation strength is considerably higher for the nanotwinned structure than for single crystal cBN, an unexpected phenomenon that challenges existing theory and understanding. We identify that this extraordinary strengthening stems from the highly anisotropic shear stress response in cBN under normal indentation pressures combined with the directional bonding configuration at the TBs of nt-cBN, which turns the weak bonding gradually into hard bonding as the deformation strain increases, giving rise to a large strain stiffening in nt-cBN [9] . This TB-dominated indentation strain-stiffening mechanism may also be applicable to other strong covalent solids. Characterization of indentation process Compared with previously studied nanograined cBN (ng-cBN) that contains only GBs with larger grain sizes (above 14 nm) [17] , [18] , the newly synthesized nt-cBN exhibits similarly high oxidation temperature and fracture toughness but much enhanced hardness (108~95 GPa versus 80~65 GPa) [6] , [18] . The fine TBs in nt-cBN are a unique structural feature distinguishing it from ng-cBN, and its extraordinary strengthening is likely driven by this new structural feature. In this work, we perform first-principles calculations (see Methods) to determine the stress–strain relation that describes the indentation process where shear and normal compressive stresses coexist beneath the indenter ( Fig. 1a ). These calculations provide crucial insights into local bond breaking mechanism that determines incipient plasticity in a crystal [23] , and the obtained ideal indentation strength sets an upper bound on material strength, which can be reached in high quality samples [24] . This approach captures essential physics in indentation tests and is especially useful in a comparative study of different materials or structures, such as nt-cBN and cBN, and in identifying the atomistic mechanisms [9] , [19] , [20] , [23] , [24] , [25] , [26] , [27] , [28] , [29] , [30] . 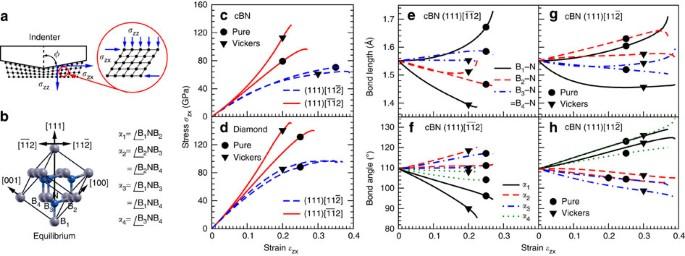Figure 1: Structural model and stress and bond-length response of cBN. (a) Sketch of indentation stress conditions. (b) The unit cell, crystalline directions and definition of bond lengths and angles of cBN. (c,d) Calculated stress–strain curves of cBN and diamond in the easyand harddirections under pure and (Vickers) indentation shear deformation. (e–h) Calculated bond lengths and angles of cBN. Figure 1: Structural model and stress and bond-length response of cBN. ( a ) Sketch of indentation stress conditions. ( b ) The unit cell, crystalline directions and definition of bond lengths and angles of cBN. ( c , d ) Calculated stress–strain curves of cBN and diamond in the easy and hard directions under pure and (Vickers) indentation shear deformation. ( e – h ) Calculated bond lengths and angles of cBN. Full size image Stress–strain relation of cubic boron nitride To understand the unexpected strengthening in nt-cBN, it is instructive to examine the stress response and deformation modes in the single crystal structure of cBN ( Fig. 1b ). We probe the stress–strain relation of cBN along its easy and hard shear directions on the weakest cleavage (111) plane [20] , [27] . In the (111) hard direction, the stress response under indentation at large strains ( Fig. 1c ) is significantly stronger than the pure shear stress, which is calculated by neglecting the normal compressive pressure beneath indenter (see Methods). But the difference between them is minimal in the (111) easy direction. Similar results are obtained for diamond ( Fig. 1d ). This intriguing contrast stems from the highly anisotropic directional bonding structure, which is common in covalent solids. In cBN the compressive stress ( σ zz ) under indentation suppresses the stretching of B 1 –N bond. It prevents the transition towards the layered graphite-like structure caused by the quick rise of the B 1 –N bond ( Fig. 1e,g ) that occurs under pure shear deformation [27] . This effect is more pronounced in the hard direction with larger reduction of the key bond length R 1 =B 1 –N and angle α 1 = ∠ B 1 NB 2 ( Fig. 1e–h ). In single crystal cBN and diamond, shear deformations in the easy and hard directions coexist under an indenter. The lower peak stress in the easy direction determines the indentation strength. The calculated values of 64.8 GPa and 97.3 GPa agree well with the measured Vickers hardness of 55 GPa and 100 GPa for cBN and diamond, respectively [6] . Stress response of nanotwinned cubic boron nitride We calculate the stress response of nt-cBN using a supercell with nine BN bilayers between neighbouring TBs (nt-cBN-9) ( Fig. 2a ), which has a TB separation of λ =1.864 nm. The (001) TB plane here is equivalent to the {111} TB plane in the cBN unit cell (see Fig. 1b ) identified in the experiment [6] . The calculated density of states and band gap in nt-cBN are almost identical to those of cBN ( Fig. 2b ), indicating low potential barriers or formation energies of TBs. The tensile results ( Fig. 2c ) indicate that the {001} and {110} planes, which have similar tensile stress peaks, are the most likely cleavage surfaces of the nanograins in nt-cBN specimen. Our calculated stress peaks under pure shear on these planes ( Fig. 2d ) are all <80 GPa. We show below that indentation causes extraordinary shear strength enhancement on both the {001} and {110} planes of nt-cBN, thus explaining the experimental results [6] . 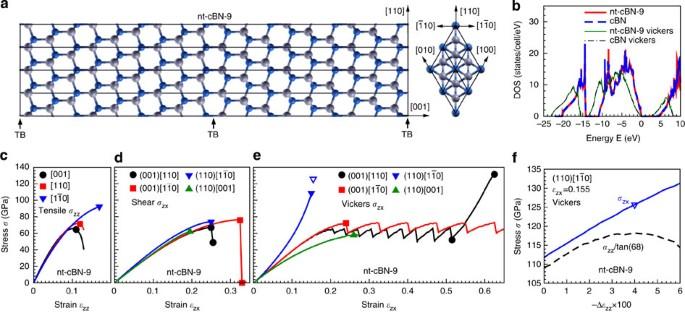Figure 2: Structural model and stress–strain relation of nt-cBN. (a) The front and side view of the supercell and crystalline directions of nt-cBN-9. (b) Calculated electronic density of states for nt-cBN-9 and cBN at equilibrium (thick lines) and under (110)(Vickers) indentation shear atε=0.1 (thin lines). (c–e) Calculated stress–strain curves of nt-cBN-9 under tensile, pure shear and (Vickers) indentation shear deformations. (f) The change of the shear and normal stress for nt-cBN-9 atεzx=0.155 as the normal compression (−Δεzz) increases after the shear stress reaches its peak indicated by the solid triangle-down symbol ine. The hollow triangle symbols in (e,f) indicate the shear stress (σzx) under the largest normal stress (σzz) at which the nt-cBN-9 structure starts to collapse. Figure 2: Structural model and stress–strain relation of nt-cBN. ( a ) The front and side view of the supercell and crystalline directions of nt-cBN-9. ( b ) Calculated electronic density of states for nt-cBN-9 and cBN at equilibrium (thick lines) and under (110) (Vickers) indentation shear at ε =0.1 (thin lines). ( c – e ) Calculated stress–strain curves of nt-cBN-9 under tensile, pure shear and (Vickers) indentation shear deformations. ( f ) The change of the shear and normal stress for nt-cBN-9 at ε zx =0.155 as the normal compression (−Δ ε zz ) increases after the shear stress reaches its peak indicated by the solid triangle-down symbol in e . The hollow triangle symbols in ( e , f ) indicate the shear stress ( σ zx ) under the largest normal stress ( σ zz ) at which the nt-cBN-9 structure starts to collapse. Full size image Figure 2e shows distinct stress patterns along two nonequivalent shear directions in the (001) plane of nt-cBN under (Vickers) indentation shear deformation: (i) a saw-teeth pattern leading to a greatly enhanced stress peak of 130 GPa in the (001)[110] direction and (ii) a periodic saw-teeth pattern in the (001) direction. These unique patterns are attributed to intriguing bond rearrangements near the TBs. To illustrate this mechanism, we show in Fig. 3 structural snapshots of nt-cBN-9 under Vickers indentation. Under the (001)[110] indentation shear, the upper half of the unit cell is deformed in the easy shear direction, while the lower half is deformed in the hard shear direction. Consequently, the stretching of atomic bonds is much larger in the upper half of the unit cell than that in the lower half. The calculations show that the most stretched bond (R 1 ) lies right next to the (middle) TB due to the stress concentration near the (middle) TB. Such stress concentration and the resulting uneven bond stretching pattern ( Fig. 3b ) are driven by the normal indentation pressure. In contrast, under pure shear deformation without the normal compressive pressure, the bond stretching is nearly uniformly distributed in the unit cell (see Fig. 4 and related discussions below). At increasing shear strain, the most stretched bond (R 1 ) breaks and rebonds in such a way that it turns the atomic layer right next to the (middle) TB from the easy direction into the hard direction (see the atomic layers enclosed by the red boxes in Fig. 3b,c ). It moves the middle TB up by one BN layer ( Fig. 3c ). This process continues until all the BN layers in the upper half of nt-cBN-9 are turned into the hard-direction alignment, leading to greatly enhanced strength ( Fig. 2e ). This is similar to the strain-stiffening effect recently discussed in inorganic crystalline solids [9] where the strengths of materials enhance greatly arising from atomic rebonding under large (indentation) structural deformations. 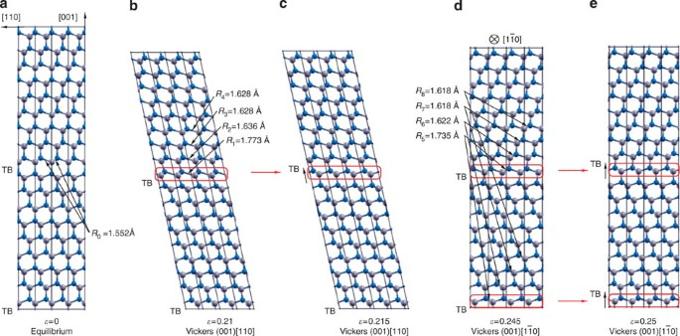Figure 3: Structural response of nt-cBN under indentation deformation. Calculated structural snapshots of nt-cBN-9 under Vickers indentation in various shear directions at (a)ε=0 at equilibrium, (b,c)ε=0.21 and 0.215 in (001)[110] direction, and (d,e)ε=0.245 and 0.25 in (001)direction pointing into the page. R1,···R8in (b,d) indicate the lengths of several most stretched bonds. Figure 3: Structural response of nt-cBN under indentation deformation. Calculated structural snapshots of nt-cBN-9 under Vickers indentation in various shear directions at ( a ) ε =0 at equilibrium, ( b , c ) ε =0.21 and 0.215 in (001)[110] direction, and ( d , e ) ε =0.245 and 0.25 in (001) direction pointing into the page. R 1 ,···R 8 in ( b , d ) indicate the lengths of several most stretched bonds. 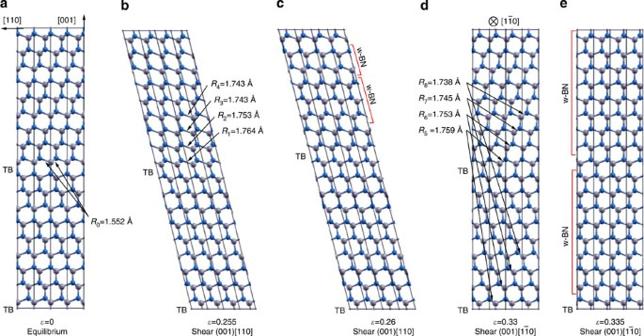Figure 4: Structural response of nt-cBN under pure shear deformation. Calculated structural snapshots of nt-cBN-9 under pure shear deformation in various shear directions at (a)ε=0 at equilibrium, (b,c)ε=0.255 and 0.26 in (001)[110] direction, and (d,e)ε=0.33 and 0.335 in (001)direction pointing into the page. R1,···R8in (b,d) indicate the lengths of several most stretched bonds. Full size image Figure 4: Structural response of nt-cBN under pure shear deformation. Calculated structural snapshots of nt-cBN-9 under pure shear deformation in various shear directions at ( a ) ε =0 at equilibrium, ( b , c ) ε =0.255 and 0.26 in (001)[110] direction, and ( d , e ) ε =0.33 and 0.335 in (001) direction pointing into the page. R 1 ,···R 8 in ( b , d ) indicate the lengths of several most stretched bonds. Full size image One notes that the opposite (001) direction is equivalent to the (001)[110] direction in nt-cBN under indentation shear deformation, except with the upper half of the atomic bonds pointing to the hard and lower half to the easy direction. And the threefold rotational symmetry on the (001) plane of nt-cBN-9 makes the six shear directions [110] , , and on the (001) crystalline plane all equivalent. They form three pairs of mutually opposing indentation strain-stiffening shear directions evenly separated by 60°. This leaves no weak or easy direction in the (001) plane under indentation shear deformation and, consequently, produces very high Vickers hardness for nt-cBN as observed in the experiment [6] . On the other hand, under the (001) indentation shear, the bond stretching patterns in the upper and lower half of nt-cBN-9 are the same ( Fig. 3d ). The most stretched bonds (R 5 ) lie next to all the TBs, and their breaking and rebonding at large strains result in a simple shift of all the TBs in the same direction without changing the overall structure ( Fig. 3e ). This produces the periodic saw-tooth stress pattern with each saw-tooth corresponding to a bond flipping event ( Fig. 2e ). We also examined structural response of nt-cBN-9 under pure shear in the (001) plane. Key structural snapshots of nt-cBN-9 under pure shear deformation in various shear directions are given in Fig. 4 . Under (001)[110] pure shear ( Fig. 4b,c ), the stretching of atomic bonds is much larger in the upper half, which points in the easy shear direction, than that in the lower half, which points in the hard shear direction, with the most stretched bonds (R 1 ,···R 4 ) evenly distributed in the upper half of the nt-cBN-9 structure. In contrast, under (001) pure shear ( Fig. 4d,e ), bond stretching in the upper and lower half of nt-cBN-9 is the same, with the most stretched bonds (R 5 ,···R 8 ) evenly distributed in the whole nt-cBN-9 cell. With further increase of the shear strain, these stretched bonds break and rebond to form various local wurtzite BN (w-BN) structures in the upper half of or the whole nt-cBN-9 cell (see Fig. 4c,e ), which have much lower shear strength. The stress in the upper half of or the whole nt-cBN-9 cell is relaxed after rebonding (see Fig. 2d ). The pure shear direction of (001) and (001) are equivalent to that of (001)[110] and (001) , except with the bonds in the lower half of or the whole nt-cBN-9 cell breaking and rebonding to form various local w-BN structures under large pure shear deformation. This leaves no hard direction on the (001) plane of nt-cBN-9 under pure shear deformation. We next analyze the shear stress response in the (110) plane. Results in Fig. 2e show that stress rises quickly along the (110) direction. Unlike the situation in cBN, the two opposing shear directions (110) and (110) in nt-cBN are both (equivalent) hard directions, and this prevents the indenter from cutting deep into sample surfaces. The (110) plane of nt-cBN is thus also expected to exhibit an unusually high indentation strength. Results in Fig. 2f show that under increasing normal compression (−Δ ε zz ) after the peak shear stress, the normal stress ( σ zz ) deviates from the relation σ zz = σ zx × tan φ ( φ =68 ° for Vickers indenter) and starts to decrease, signalling a compressive bond collapse mechanism in nt-cBN (see Methods), rather than the usual shear breaking mechanism under pure shear strain [27] . The shear stress ( σ zx ) under the largest normal stress ( σ zz ) reaches 126 GPa, which is driven by the same mechanism for the indentation strengthening of cBN in its hard direction. The B 1 –N and B′ 1 –N′ bonds in nt-cBN on the two sides of a TB tilt towards each other ( Fig. 5a ), providing a stronger resistance to the normal pressure in the [110] direction, and producing a large contraction of the key bond lengths and angles ( Fig. 5b,c ), similar to the results shown in Fig. 1e,f . 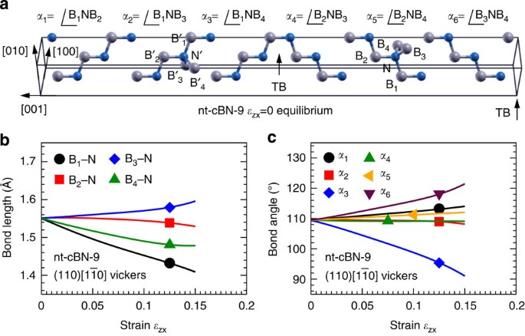Figure 5: Structural model and response of nt-cBN under indentation. (a) The unit cell, crystalline directions and definition of bond lengths and angles of nt-cBN-9. (b,c) Calculated bond lengths and angles of nt-cBN-9 under the (110)(Vickers) indentation shear deformation. Figure 5: Structural model and response of nt-cBN under indentation. ( a ) The unit cell, crystalline directions and definition of bond lengths and angles of nt-cBN-9. ( b , c ) Calculated bond lengths and angles of nt-cBN-9 under the (110) (Vickers) indentation shear deformation. Full size image To test the robustness of the TB-dominated strength enhancement (indentation strain stiffening) mechanism, we examined nt-cBN structures with different number of defective TBs and larger TB separation size and obtained nearly identical stress patterns and indentation strength (see Fig. 6a–g ), which suggests that our calculated results are insensitive to such variations of TBs, especially the defective TBs, which were pointed out to exist in the nt-cBN specimen [31] and suspected to reduce its hardness compared with the nt-cBN with ideal sharp TBs. The nanotwin separation of nt-cBN-18 ( Fig. 6g ) is λ =3.728 nm, close to the average nanotwin separation ( λ =3.8 nm) of the nt-cBN specimen synthesized in the experiment [6] . The TB-dominated strengthening mechanism also applies to other strong covalent solids that share the same generic structural characteristics. In particular, we obtained nearly identical stress patterns for a nanotwinned diamond nt-Dia-9 structure that exhibits a record-setting high indentation strength of 150 GPa on its main (001) and (110) easy cleavage planes (see Fig. 6h ). 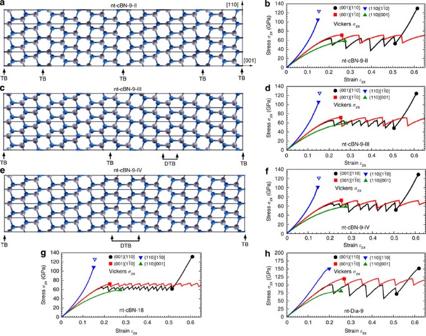Figure 6: Additional structural models and stress response of nt-cBN and nt-diamond. The front view and calculated stress–strain curves under various (Vickers) indentation shear deformations for (a,b) a nt-cBN-9 supercell with four twin boundaries (TBs) (nt-cBN-9-II), (c,d) a nt-cBN-9 supercell with two TBs and one defective TB (DTB) made of two wurtzite BN (w-BN) layers (nt-cBN-9-III), and (e,f) a nt-cBN-9 supercell with one TB and one DTB made of three w-BN layers (nt-cBN-9-IV). (g,h) The calculated stress–strain curves of nt-cBN-18 and nt-Dia-9 under various (Vickers) indentation shear deformations. The hollow triangle symbols in (b,d,f,g) indicate the shear stress (σzx) in the (110)shear direction under the largest normal stress (σzz) at which the corresponding nt-cBN structure starts to collapse (see the related discussion onFig. 2f). Figure 6: Additional structural models and stress response of nt-cBN and nt-diamond. The front view and calculated stress–strain curves under various (Vickers) indentation shear deformations for ( a , b ) a nt-cBN-9 supercell with four twin boundaries (TBs) (nt-cBN-9-II), ( c , d ) a nt-cBN-9 supercell with two TBs and one defective TB (DTB) made of two wurtzite BN (w-BN) layers (nt-cBN-9-III), and ( e , f ) a nt-cBN-9 supercell with one TB and one DTB made of three w-BN layers (nt-cBN-9-IV). ( g , h ) The calculated stress–strain curves of nt-cBN-18 and nt-Dia-9 under various (Vickers) indentation shear deformations. The hollow triangle symbols in ( b , d , f , g ) indicate the shear stress ( σ zx ) in the (110) shear direction under the largest normal stress ( σ zz ) at which the corresponding nt-cBN structure starts to collapse (see the related discussion on Fig. 2f ). Full size image We have identified a twin-boundary dominated mechanism for extraordinary strengthening in classic reverse Hall–Petch regime in nt-cBN. It expands the scope of our understanding of microstructural size control on materials strength. Such new insights into the atomistic mechanisms for incipient plastic deformation in nanostructured covalent materials may facilitate other large-scale modelling, such as ab initio -MD or ab initio -finite element simulations, of stress response and plasticity in these promising materials. The present work can be extended to other strong covalent solids that share the directional and anisotropic bonding characteristics. First-principles calculations The ideal strength calculations were performed using the VASP code (See the web site: http://www.vasp.at/ ), adopting the projector augmented wave potentials [32] , the local-density-approximation with the exchange-correlation functional of Ceperley and Alder [33] as parametrized by Perdew and Wang [34] and a plane-wave basis set. A 500 eV energy cutoff, and a 10 × 10 × 2 and 10 × 10 × 1 Monkhorst–Pack k-point grid [35] were used for nt-cBN-9 and nt-cBN-18, respectively, with the unit cell given in Fig. 5a ; (a 10 × 10 × 10 k-point grid is used for cBN with the unit cell given in Fig. 1b ). The energy, stress and force convergence are 1 meV per atom, 0.1 GPa and 0.001 eV Å −1 , respectively. To simulate the indentation process with first-principles calculations, we consider a biaxial stress distribution beneath an (Vickers) indenter with a shear stress and a normal compressive stress (pressure) component (see Fig. 1a ), which captures the main characteristic of the indentation process and is more realistic compared with the previous pure ideal shear strength calculations that neglect the effect of normal compressive pressures [9] , [19] , [20] , [23] , [24] , [25] , [26] , [27] . The contact force between the indenter face and the specimen is decomposed into two components: F x parallel to the specimen surface and F z perpendicular to the surface. These force components project onto the same contact area and produce a pure shear stress component σ zx = F x / A z and a normal compressive stress (pressure) component σ zz = F z / A z where A z is the projected area under the indenter. They are related by σ zz / σ zx =tan φ , where φ =68° is the the centerline-to-face angle of a Vickers indenter. The quasistatic ideal indentation strength and relaxed loading path were determined using a recently developed method [28] , [29] , [30] , in which the lattice vectors of the unit cell of the crystal structure were incrementally deformed in the direction of the applied shear strains with an incremental strain step of Δ ε =0.005. At each step, the applied shear strain, say ε zx , is fixed which determines the calculated shear stress σ zx , while the other five independent components of the strain tensors and all the atoms inside the unit cell were simultaneously relaxed until the following conditions are met: (i) the compressive pressure ( σ zz ) beneath the indenter normal to the chosen shear deformation plane reaches a specified value (that is, σ zz = σ zx tan φ ), (ii) all the other four components (that is, σ xx , σ yy , σ yx and σ zy ) of the Hellmann–Feynman stress tensor are negligibly small (<0.1 GPa) and (iii) the force on each atom becomes negligible (<0.001 eV Å −1 ). The shape of the (deformed) unit cell, the positions of the atoms and the relation between the shear stress σ zx and shear strain ε zx are determined completely at each step by this constrained atomic relaxation, including the effect of the normal compressive pressure σ zz . The peak stress in a given indentation shear direction determines the stress at which the crystal structure starts to destabilize. Different indentation shear deformation directions are calculated to determine the indentation strength of the crystal structure. The present method is versatile in its ability to simulate various shear deformation modes that are useful for the analysis of the indentation strength of the crystal structure. When we set φ =0 (thus σ zz =0) in the calculation, it is equivalent to requiring that all the five stress components (except σ zx ) become negligible during the structural relaxation, which is the relaxation procedure widely used in the calculations of pure ideal shear stresses that neglect the effects of the normal compressive pressure and geometry (indenter angles) of the indenter [9] , [19] , [20] , [23] , [24] , [25] , [26] , [27] . We can also set both ε zx and ε zz fixed in the calculation procedure so that both stresses σ zx and σ zz are obtained independently for a given set of ε zx and ε zz . Such calculations were performed in the present work to obtain the results presented in Fig. 2f , which show that as the shear strain ε zx increases, the normal stress σ zz deviates from the relation σ zz = σ zx tan φ required for the indentation process no mater how much the structure is compressed. When σ zz starts to decrease after reaching its peak as the compression continues, it indicates a collapse of the structure by the normal compressive pressure during the indentation process. How to cite this article: Li, B. et al . Large indentation strain stiffening in nanotwinned cubic boron nitride. Nat. Commun. 5:4965 doi: 10.1038/ncomms5965 (2014).